CDK6 inhibits white to beige fat transition by suppressing RUNX1 Whereas white adipose tissue depots contribute to the development of metabolic diseases, brown and beige adipose tissue has beneficial metabolic effects. Here we show that CDK6 regulates beige adipocyte formation. We demonstrate that mice lacking the CDK6 protein or its kinase domain (K43M) exhibit significant increases beige cell formation, enhanced energy expenditure, better glucose tolerance, and improved insulin sensitivity, and are more resistant to high-fat diet-induced obesity. Re-expression of CDK6 in Cdk6 −/− mature or precursor cells, or ablation of RUNX1 in K43M mature or precursor cells, reverses these phenotypes. Furthermore, RUNX1 positively regulates the expression of Ucp-1 and Pgc1α by binding to proximal promoter regions. Our findings indicate that CDK6 kinase activity negatively regulates the conversion of fat-storing cells into fat-burning cells by suppressing RUNX1, and suggest that CDK6 may be a therapeutic target for the treatment of obesity and related metabolic diseases. Obesity has long been known to be the most important risk factor for the development of type II diabetes and other metabolic diseases. In rodents and humans, fat is deposited as energy storage in white adipose tissue (WAT), whereas fat is consumed to produce heat in the mitochondria-rich brown adipose tissues (BAT). As a thermogenic tissue, inducible-brown adipocytes (also called beige or brite cells) are found sporadically in WAT of adult animals with similar features as classical brown adipocytes but originate from a non-myf5-derived cell lineage, likely developed from the progenitor cells residing in the stromal vascular fraction (SVF) of white adipose depots. Importantly, the activation of beige cells is associated with a protection against obesity and metabolic diseases in rodent models and correlated with leanness in human [1] , [2] . Cold-induced activation of sympathetic nervous system (SNS) was previously widely believed to be the primary or only physiological signal to activate BAT/beige cells development and function, which can be mimicked by treating mice with β3-adrenergic (β3-AR) activators [3] . In addition, many genes and pathways that drive brown-fat-like thermogenesis in murine white fat have now been identified. In particular, the discovery of circulating factors such as exercise-induced cytokine (FGF-21) [4] and mytokine (Irisin) [5] provide a variety of promising therapeutic targets for metabolic diseases. However, while at first it may seem plausible to treat humans with β3-AR agonists, differences between rodent and human receptor physiology lead to significant off target effects [6] , [7] . In turn, this has halted the development of β3-AR agonists as a viable treatment for obesity-related metabolic diseases. Nevertheless, the challenges facing long-term maintenance of regular exercise and cold exposure abound, due to natural human tendency for thermal comfort as well as modern-day time constraints. Thus, in face of the imminent epidemic, there is an urgent need for a new therapeutic target to attain weight control and to improve the obesity-related metabolic profile. Cyclin-dependent Kinase 6 (CDK6) plays an important role in proliferation and differentiation [8] . Although regulation of cell cycle is deemed to be the primary function of CDK6 [9] , it also acts in a cell cycle-independent manner, as evidenced by binding and promoting the degradation of RUNX1 (also known as AML1) [10] . As a member of the Runt-related transcription factors, RUNX1 recognizes a specific DNA sequence, which upon binding, activates or represses the transcription of several downstream genes [11] . However, the molecular roles that CDK6 and RUNX1 play in obesity and its associated metabolic diseases remains largely unexplored. Employing our defined Cdk6 mouse models and in vitro differentiation assay, we have observed that the loss of either CDK6 ( Cdk −/− ) or its kinase domain ( K43M ) results in white fat browning, enhanced energy expenditure, improved glucose tolerance and insulin sensitivity, and resistance to high-fat diet (HFD)-induced obesity (DIO). Importantly, recovery of CDK6 expression or ablation of Runx1 reversed this metabolic phenotype. Therefore, targeting CDK6 may be a therapeutic strategy to treat obesity and its related metabolic diseases. CDK6 responds to changes in nutritional status To explore the function of CDK6 in adiposity, we first determined the expression of CDK6 protein in adipose tissues. In male and female mice, CDK6 was expressed in both BAT and WAT, e.g. inguinal WAT (iWAT) and epididymal WAT (eWAT), respectively (Supplementary Fig. 1a ). Similar to leptin, a protein produced by fatty tissue and considered to regulate fat storage, CDK6 mRNA and protein were selectively up-regulated in iWAT and eWAT but not in BAT in C57BL/6J mice under an HFD compared to the mice under a normal chow diet (NCD) (Supplementary Fig. 1b, c ). Furthermore, CDK6 protein level was also higher in mice that fasted overnight compared to the mice on an NCD (Supplementary Fig. 1d ). Taken together, these data indicate that CDK6 responds to changes in nutritional status. K43M mice are resistant to HFD-induced obesity To understand the functional relevance of CDK6 in obesity and its related diabetes, we utilized CDK6 knockout and knockin mice [12] , [13] . We produced genetically distinct animals by introducing a LoxP-flanked transcriptional STOP cassette (LSL cassette) into intron 1 of the Cdk6 gene adjacent to the intact or mutant exon1. In the presence of the LSL cassette, CDK6 expression is prevented, which results in a null allele named: Cdk6 −/− (KO) , or WT-LSL , or K43M-LSL (Supplementary Fig. 1e ). Upon excision of the cassette by germline expression of Cre recombinase (Nestin-CRE), the CRE-reactivated wild-type (referred to as WT hereafter) or the mutant alleles express either WT or mutant protein (Supplementary Fig. 1f ), respectively, from the endogenous locus with intact regulatory controls, specifically, the knockin mutant with a catalytically inactive kinase domain, CDK6 K43M (K43M) [13] . The significance of this particular mutant is that Lys 43 residue is highly conserved across all eukaryotic kinases and represents one of three residues forming a triad of catalytic residues involved in ATP phosphate orientation and Mg2+ coordination [14] , [15] . Therefore, expression of the K43M mutation is a powerful genetic model equivalent to pharmacological inhibition of CDK6 kinase activity. To investigate if loss of CDK6 kinase activity alters the metabolic physiology of the mice, we first subjected wild-type ( WT ) and K43M mice to either NCD or an HFD (starting at 4-week-old) over a 14-week period. Both male and female (data not shown) K43M mice displayed increased resistance to weight gain under NCD and HFD (Fig. 1a, b , Supplementary Fig. 2a ). To help elucidate the underlying mechanism governing protection against DIO, we isolated different fat pads and tissues of 12-week-old (Supplementary Fig. 2c, d ) and 18-week-old (Fig. 1c, d ) mice, respectively, and measured their weighs relative to the whole-body weights of the mice. We observed that K43M mice had significantly decreased fat pad mass (~1.5- to 4-fold reduction compared with WT ) in all WAT depots analyzed, including iWAT, eWAT, and perirenal (Peri-R) compartments, which were consistent with decreased adiposity assessed using NMR (Supplementary Fig. 2a, b ). By contrast, interscapular BAT depots were not significantly different in weight between WT and K43M mice (Fig. 1c, d and Supplementary Fig. 2e ). In addition, no significant mass changes were observed in the liver of WT and K43M mice under NCD and HFD (Fig. 1c, d ). Collectively, these results show that loss of CDK6 kinase activity systemically in mice protects from DIO. Fig. 1 Loss of CDK6 kinase activity in mice leads to an improved metabolic profile. a , b Body weight of age-matched male mice on NCD ( a ) or HFD ( b ) for a 14-week observation time. HFD commenced at 4 weeks of age. c , d Mass of various fat pads was normalized to body weight of male mice on NCD ( c ) or HFD ( d ) at 18 weeks of age. No significant changes were observed in the masses of BAT and livers between WT and K43M mice under NCD and HFD. e , f GTT after 14 weeks on NCD ( e ) or HFD ( f ). g , h ITT after 14 weeks on NCD ( g ) or HFD ( h ). For a – h , data shown are mean ± S.E. ( n = 10 for each group), * p < 0.05, t -test, vs WT . See also Supplementary Figs. 2 and 3 Full size image K43M mice exhibited improved GTT and ITT We next evaluated whether K43M mice exhibited an improved metabolic profile by conducting intraperitoneal glucose- and insulin-tolerance tests (IP-GTT and IP-ITT, respectively). Compared to their WT littermates, K43M mice fed on both NCD and HFD displayed rapid clearance and resulted in lower blood glucose concentrations after glucose (Fig. 1e, f ) and insulin (Fig. 1g, h ) injection, suggesting that genetic disruption of CDK6 improves blood glucose tolerance and insulin sensitivity. Loss of CDK6 kinase activity leads to white fat browning Under NCD, both male (Fig. 2 ) and female (data not shown) K43M mice were found on dissection to have browner appearance in various fat pads, such as posterior-subcutaneous (Fig. 2a ) and iWAT (Fig. 2b ), than their WT counterparts. The size of adipocytes in K43M mice were smaller (Fig. 2c ) but the brown-type features of iWAT were evidenced by presence of much more abundant multilocular UCP-1 + beige adipocytes in iWAT (Fig. 2d ). By contrast, despite reduced fat pad mass and smaller cell sizes, K43M and WT mice had similar appearance with comparable UCP-1 + staining in eWAT (Fig. 2e–h ), suggesting that the underlying mechanisms governing the homeostasis of sWAT and visceral adipose tissue (VAT) of K43M mice were different. Consistently, BAT-specific genes Ucp-1 , Pgc-1α , Cidea , and Prdm16 were expressed at significantly higher levels in iWAT (Fig. 2i ) but not in eWAT (Fig. 2j ) of K43M mice compared to WT . In contrast, the WAT-specific genes including Ap2 , Adiponectin (AdipoQ) , and Leptin were expressed at comparable levels in iWAT and eWAT (Fig. 2i, j ) from both K43M and WT mice. Furthermore, iWAT but not eWAT of K43M mice had higher expression of mitochondria DNA (mtDNA) than that of WT mice (Fig. 2k ). In parallel with mRNA levels, UCP-1 and PGC-1α, two factors contributing to leanness in various mouse models [16] , were selectively expressed at higher levels in iWAT, but not eWAT of K43M mice as compared to WT mice (Fig. 2l , Supplementary note), suggesting enhanced beige cells in iWAT depots. However, mass and cell size in BAT (Supplementary Fig. 2e–g ) were comparable between WT and K43M mice. Moreover, although BAT-specific genes were also marginally, yet significantly, increased in the BAT (~1.8- to 2.3-fold) (Supplementary Fig. 2h ) of K43M mice, no significant differences were noted in CDK6, PGC-1a, and UCP-1 protein levels between WT -BAT and K43M -BAT mice under NCD (Supplementary Fig. 2i ). Taken together, these data suggest that increased white fat browning, rather than an overall reduced WAT adipogenesis, may underlie the reduced fat pad mass in K43M mice under NCD. Fig. 2 Loss of CDK6 kinase activity in mice induced white fat browning. a , e Appearance of male posterior-subcutaneous WAT (sWAT) ( a ), and dorsal view of NCD-fed WT and K43M mice ( e ), emphasized with blue squares and arrows. b , f Appearance of a close view of the iWAT ( b ) and eWAT ( f ) from the mice indicated. c , g Representative light microscopic images of H&E-stained sections of iWAT ( n = 6) and eWAT ( n –6) from male mice indicated (scale bars: 100 μm). d , h Representative images of UCP-1 immunohistochemical staining ( n = 6) of iWAT and eWAT from mice indicated at 18 weeks of age (scale bars: 100 μm). i , j Relative mRNA expression levels of BAT-specific markers ( Ucp-1 , Pgc-1α , Cidea , and Prdm16) and WAT-specific markers ( Ap2 , adiponectin-AdipoQ , and Leptin ) of iWAT ( i ) and eWAT ( j ) tissues from WT and K43M mice. Data shown are mRNA fold change normalized to the control WT , which is arbitrarily set to 1 unit. k Relative expression levels of mtDNA of eWAT and iWAT from WT and K43M mice. Data shown are fold change of mtDNA compared to control. For i and j , * p < 0.05, vs WT ( n = 6), t -test. i Immunoblots of the indicated protein levels in iWAT and eWAT from 50 μg of cell lysates of WT and K43M mice at 18 weeks of age. α-Tubulin is used as an internal loading control. See also Supplementary Figs. 2 and 3 Full size image Under the same experimental condition, we also observed that the RUNX1 protein, a downstream target of CDK6 [17] , [18] was increased in iWAT but not in eWAT of K43M adipocytes in comparison to WT controls (Fig. 2l ). However, the levels of Runx1 mRNA were comparable (Supplementary Fig. 2j ), thereby ruling out a transcriptional effect of K43M on RUNX1 levels. Together with the known essential functions of RUNX1 in many biological programs related to development [19] , we hypothesized that RUNX1 may be involved in the process of white fat browning in iWAT of K43M mice. Under HFD, a ~3- to 80-fold induction of BAT-specific genes (Supplementary Fig. 3g ) and a ~1.5- to 3-fold suppression of WAT-specific genes (Supplementary Fig. 3h ) were observed in iWAT of K43M mice vs those in WT mice. RUNX1 protein was also increased in the iWAT of K43M compared to WT controls (Supplementary Fig. 3i ). Together, these data suggest that under NCD, the gross reduction of sWAT pad mass in K43M mice resulted from a partial replacement of white fat with beige cells. Under HFD, however, both increased white fat browning and reduced WAT adipogenesis in K43M mice might account for the reduced adiposity in K43M mice. K43M mice have increased energy expenditure A physiological hallmark of beige cells is their highly active metabolism coupled to thermogenesis, similar to that featured in classical brown fat cells [20] . To determine if increased browning in K43M mice correlates with increased caloric intake as well as thermogenesis, we examined the food consumption and body temperature of mice under different conditions. As expected, K43M mice had significantly more food intake (4.25 ± 0.05 g/day) than WT mice (3.6 ± 0.09 g/day) (Fig. 3a ) and elevated body temperature compared to WT mice at room temperature (Fig. 3B , RT). Robust differences were apparent after cold exposure: the body temperature of WT mice was significantly lower than their K43M counterparts by 0.28 °C (1-day, p = 0.03), 0.67 °C (2-day, p = 0.02), and 0.90 °C (3-day, p = 0.03), respectively (Fig. 3c ). Upon dissection, K43M mice were found to have browner appearance in iWAT than their WT counterparts but comparable appearance on BAT (Supplementary Fig. 4a–c ). Compared with WT -iWAT, the magnitude of the increment in Ucp-1 gene and protein expression in K43M -iWAT was much smaller (Supplementary Fig. 4d, e ) than those in RT (Fig. 2i, l and Supplementary Fig. 4g ). It is noteworthy that RUNX1 protein but not the mRNA level in K43M-iWAT was also enhanced under cold exposure (Supplementary Fig. 4d, e ). However, the expressions of Cdk6 gene and protein were comparable between WT and K43M mice. These results indicate that increased white fat browning in K43M mice is reflected by a significantly higher body temperature and thus more adaptive than WT mice to cold-induced thermogenesis. Fig. 3 Loss of CDK6 kinase activity in mice leads to increased food intake, body temperature, adaptability to cold exposure and energy expenditure. a Bar graphs demonstrating food intake of age-matched male WT and K43M mice at 18 weeks of age. b , c Core body temperature of male mice at room temperature ( b , RT) or at 4 °C ( c ) for up to 72 h ( n = 6 per group). d Energy expenditure (EE) was calculated based on the formula below: EE = (3.815 + 1.232 × RER) x VO 2 /lean mass (g). For a – d , data are expressed as mean ± S.E., * p < 0.05, vs WT , t -test. e – h , Oxygen consumption (VO 2 ) (e, f) and CO 2 production (VCO 2 ) (g, h) from metabolic cages of male WT and K43M mice on NCD ( n = 6) in 12 h light and dark phases. VO 2 and VCO 2 were normalized by lean mass. * p < 0.05, vs WT , log-rank tests. i Bar graphs displaying mean Respiratory Exchange Ratios (RER) over 24-h period. RER was calculated as the volume of CO 2 vs the volume of oxygen (VCO 2 /VO 2 ). j Physical activity of male WT and K43M mice in the periods of 12 h light and 12 h dark phase. k Ex vivo oxygen consumption of iWAT homogenates from different WT and K43M mice. Data are expressed as mean ± S.E., * p < 0.05, vs WT , t -test Full size image To further investigate the mechanism underlying the difference in reduced adiposity in 18-week-old K43M mice, we monitored the metabolic activities of these mice by using metabolic cages. NCD-fed K43M mice had increased energy expenditure during the three-day observation period (Fig. 3d ), as indicated by significantly greater O 2 consumption (Fig. 3e, f , dark phase) and greater CO 2 production (Fig. 3g, h , dark phase) than WT controls during the nocturnal phase. Importantly, there is no measurable difference in the respiration exchange ratio (RER) and physical activity between WT and K43M mice (Fig. 3i, j ). These data indicate that the reduced adiposity in K43M mice might be caused by an increase in energy expenditure rather than in physical activity. Lean mass is mainly composed of skeletal muscle, a major contributor to resting and exercise-induced energy expenditure [21] . Undetectable CDK6 protein in skeletal muscle (Supplementary Fig. 1a ) prompted us to focus on the contribution of fat tissues to energy expenditure. For this purpose, we have measured energy expenditure directly on iWAT but not the skeletal muscle of different mutant mice by using the Clark electrode to further confirm that the adipose tissues indeed contribute to the increased energy expenditure in K43M mice. When measuring the respiration rate of freshly minced fat tissue, the O 2 consumption of iWAT was increased significantly in K43M mice compared to that in WT mice (Fig. 3k ), indicating that the adipose tissues indeed contribute to the increased energy expenditure in K43M mice. However, it is unknown at present whether CDK6 contributes to the energy expenditure in skeletal muscle. Collectively, these results demonstrate that loss of CDK6 kinase activity in mice results in increased thermogenic function through elevation of energy expenditure, which may account for more adaptability in response to a cold exposure and for protection against HFD-induced obesity. SNS activation is not the major cause of white fat browning The brown appearance of WAT in K43M mice (germline) could, in principle, be mediated by activation of β–adrenergic receptors [22] , targets of the catecholamines. The loss of CDK6 function in adipocytes could result in a generalized stress response (increased adrenergic stimulation) that then indirectly results in browning of iWAT, along with increased energy expenditure and all of the other phenotypes observed in Cdk6 mutant mice. In rodents, exposure to cold stimulates the sympathetic nerve system (SNS) to biosynthesize the tyrosine hydroxylase (TH) [23] , the rate-limiting enzyme in the synthesis of noradrenaline [24] , and then release more adrenaline [25] , [26] , which increases Ucp-1 expression in WAT [27] . To examine directly if white fat browning is due to activation of SNS, firstly, we exposed mice to RT or cold environments (4 °C) with or without inhibition of noradrenaline synthesis. To achieve this, mice were treated with α-methyl- p -tyrosine (α-MPT), a competitive specific inhibitor of TH [23] , [24] , for 24 h [25] . We then examined the effects of the treatments on Ucp-1 expression in iWAT. Consistent with previous studies [23] , [25] , [27] , cold stimulation markedly enhanced TH and Ucp-1 in WT- iWAT (Supplementary Fig. 4f, g ), but this enhancement was clearly reversed with α-MPT administration in WT mice. In contrast, the magnitudes of increment in TH and Ucp-1 gene expression in K43M -iWAT after cold stimulation were much smaller (Supplementary Fig. 4f, g ) than those in WT- iWAT, and the expression of UCP-1 protein was comparable between K43M mice with or without α-MPT administration (Supplementary Fig. 4h ) at RT. These finding indicate that SNS involvement in the regulation of UCP-1 expression in WT mice, but not the major determinant in K43M mice. Therefore, the WAT browning observed in K43M mice is not chiefly mediated by activation of β-adrenergic system. Cell-autonomous effect of CDK6 on white fat browning The brown appearance of WAT in K43M mice could be a direct conversion from mature white adipocytes. To address this question, we crossed Cdk6 −/− or K43M-LSL mice with Adiponectin-Cre (Adipoq-Cre) mice (Supplementary Fig. 5a ), which express CRE in mature adipocyte [28] within WAT and BAT. The resultant mice are named WT- A and K43M- A for re-expression of CDK6 or expression of K43M proteins in mature adipocytes. DNA recombination and Cre expression in adipocytes of the resultant mice were confirmed by PCR (Supplementary Fig. 5b ) [13] . Immunoblot analysis demonstrated that the levels of CDK6/K43M expression in WT-A and K43M-A mice were about 50–60% of WT (Supplementary Fig. 5c ), which suggests that Adipoq-Cre elicited partially penetrant recombination in mature adipocytes and/or no observable recombination in the SVF [29] of white adipose depots where the beige cell progenitors reside. Consistently, no CDK6 protein in other tissues such as thymocytes (Supplementary Fig. 5d ) was detected in WT-A and K43M-A mice. In line with previous studies [29] , [30] , WT-A and K43M-A mice were born at the expected Mendelian frequency, and display fertility with normal development. They have comparable body lengths as WT and KO mice (Supplementary Fig. 5e ). Similar to K43M mice, KO and K43M-A mice ate more than WT mice, whereas WT and WT-A mice had similar food intake each day (Supplementary Fig. 5f ). We found that re-expression of CDK6 in mature adipose cells of WT-A mice reversed the browning of WAT, indicating that CDK6 negatively regulates white fat browning in a cell-autonomous manner, whereas expression of the inactive kinase ( K43M-A ) in mature adipocytes on a null background preserves the K43M or null phenotype (Fig. 4a–d ). Consistently, the BAT-specific genes were expressed at higher levels in iWAT of KO or K43M-A mice compared to controls under both NCD and HFD, which is reflected, to a similar degree, as K43M vs WT (Fig. 4e and Supplementary Fig. 3g ). A number of these genes are also modestly but significantly increased in eWAT (Supplementary Fig. 3e ) of KO and K43M-A mice. However, immunoblot analysis confirmed the higher expression of UCP-1, PGC-1α, and RUNX1 (Fig. 4f , lanes 1–4, Supplementary note) in iWAT but not in eWAT of KO and K43M-A mice (Fig. 4f , lanes 6–9, Supplementary note). By contrast, Ap2 and AdipoQ were comparable between KO/K43M-A and WT-A mice (Supplementary Fig. 3f ), as in K43M -iWAT (Fig. 2i ) under NCD, but reduced significantly under HFD (Supplementary Fig. 3h ). Leptin , however, was expressed at significantly lower levels in iWAT of KO/K43M-A under both NCD and HFD (Supplementary Fig. 3f, h ). All gene expression levels were comparable between WT-A and WT cells (Fig. 4e and Supplementary Fig. 3e–h ). Importantly, adipose-specific re-expression of CDK6 significantly reversed the increased oxygen consumption of iWAT observed in KO mice, whereas K43M-A mice recapitulated KO mice in terms of oxygen consumption (Fig. 4g ). Therefore, re-expression of CDK6 in mature adipocytes can reverse the phenotypes observed in KO mice, and adipose-specific expression of K43M can recapitulate the phenotypes observed in KO/K43M mice. Fig. 4 Re-expression of CDK6 in mature adipocytes of KO mice reverses white fat browning. Loss of kinase activity in mature adipocytes preserves the effect of loss of kinase activity in germline on white fat browning. a Appearance of male (18 weeks of age) posterior-sWAT of NCD-fed WT , WT-A , KO , and K43M-A , emphasized with blue squares and arrows. b Appearance of isolated iWAT from the mice indicated in a . c Representative light microscopic images of H&E-stained sections of iWAT ( n = 6) from male (18 weeks of age) mice indicated in a (scale bars: 100 μm). d Representative images of UCP-1 staining ( n = 6) of iWAT from mice indicated at 18 weeks of age (scale bars: 100 μm). e Relative mRNA expression levels of BAT-specific markers ( Ucp-1 , Pgc-1α , Cidea , and Prdm16) of iWAT under NCD. Data shown are mRNA fold change normalized to their respective controls, WT or WT-A . * p < 0.05, n = 6, t -test, comparing experimental group vs its control. f Immunoblots of the indicated protein levels in iWAT and eWAT from 50 μg of cell lysates. Twenty micrograms of cell lysates of BAT was used as a positive control for UCP-1 and PGC-1α, and α-tubulin was utilized as an internal loading control. g Ex vivo oxygen consumption of iWAT homogenates from mice. Data are expressed as mean ± S.E., * p < 0.05, n = 6, vs WT , t -test. ✢ p < 0.05, n = 6 vs KO , t -test. See also Supplementary Figs. 3 and 5 Full size image Cell-autonomous effect of CDK6 on GTT and ITT To check whether browning of WAT in K43M-A mice elicits the same advantageous metabolic effects as K43M mice, we fed age-matched male K43M-A together with WT , KO , and WT-A mice a NCD or a HFD for 14 weeks starting at 4 weeks of age. KO and K43M-A mice had similar body weight under both diets, exhibiting significantly reduced body weight on both NCD (Fig. 5a ) and HFD (Fig. 5b and Supplementary Fig. 3b ), compared to WT-A mice. Re-expression of CDK6 in mature adipocytes in WT-A mice restored the body weight completely under HFD but only partially under NCD compared to WT mice during the observation period (Fig. 5a, b ), suggesting that the effects of CDK6 on the development of other tissues such as thymocytes, hematopoietic stem progenitors [12] , [13] and progenitors of adipocytes might account for the baseline body weight difference between WT and WT-A mice fed with NCD. Fig. 5 Re-expression of CDK6 in mature adipocytes reversed the beneficial metabolic effects observed in KO mice, whereas re-expression of kinase dead CKD6 recapitulates this metabolic profile. a , b Body weight of age-matched male mice on NCD ( a ) or HFD ( b ) for 14-week observation time. HFD started at age of 4 weeks. c , d GTT after 18 weeks on NCD ( c ) or HFD ( d ). e , f ITT after 18 weeks on NCD ( e ) or HFD ( f ). g , h Mass of various fat pads was normalized to body weight of male mice on NCD ( g ) or HFD ( h ) at age of 18 weeks. No significant changes were observed in the masses of BAT and livers in those mice under NCD and HFD. For a – h , data are expressed as mean ± S.E. ( n = 10 for each group), * p < 0.05, t -test, vs WT-A . See also Supplementary Fig. 3 Full size image Similar to K43M mice with a germline mutation, K43M-A and KO mice displayed better glucose tolerance (Fig. 5c, d ), more sensitivity to insulin (Fig. 5e, f ), and drastically reduced fat pad masses (Fig. 5g, h and Supplementary Fig. 3d ), ranging from ~2- to 3.6-fold reduction in different fat pads, compared to those of WT-A mice. Consistent with reduced weight gain observed under NCD, WT-A had slightly but significantly reduced fat pad masses in various depots compared to those of WT mice, ranging from ~1.3- to 1.6-fold reduction, suggesting re-expression of CDK6 in mature adipocytes only partially rescued the defect of KO mice in WAT development. Together, these data suggest that adipose-specific re-expression of CDK6, but not K43M, reverses the beneficial metabolic effects observed in KO mice, indicating that the CDK6 kinase activity regulates metabolic homeostasis in a cell-autonomous manner. But it remains to be seen if only adipocyte-specific loss of CDK6 or kinase activity imparts the observed effects on the metabolic profile. Loss of CDK6/kinase activity increases beige cells in vitro The brown appearance of WAT in K43M mice (germline) could be a direct (cell-autonomous) consequence of loss of CDK6 kinase activity on specification and/or differentiation from beige precursors. In order to confirm that the observed phenotypes are indeed due to cell-autonomous adipocyte browning, we sought to determine if ablation of CDK6 kinase activity in vitro promotes differentiation towards brown-like adipocytes using mouse primary adipose derived stem cells (ADSCs) from the SVF of adipose tissue. The confluent primary ADSCs isolated from iWAT of WT , KO , or K43M mice were stimulated with brown- or white fat inducers for 7 days. With BAT inducers, ADSCs derived from K43M or KO mice turned into brown-like adipocytes (Fig. 6a, e, f ), but had defects to differentiate into WAT in the presence of WAT inducers (Fig. 6b, g ), as demonstrated by Oil Red O (ORO) staining (Fig. 6a, b, d ) as well as the increased BAT markers and reduced expression of WAT markers (Fig. 6e–g ). Consistently, KO and K43M cells contain a greater number of mitochondria than WT cells, as determined by MitoTracker staining, a cell-permeable probe used to label mitochondria (Fig. 6c ). Re-expression of CDK6 in KO cells (Fig. 6f , lane 3) after retroviral infection with MigR1-GFP-CRE [17] reversed advantageous in BAT-like differentiation (Fig. 6a, c, e, f ) and the defect in WAT differentiation (Fig. 6b, d, g ). Together, these data suggested that the absence of CDK6 kinase activity restricts precursors from executing WAT adipogenic programs in a cell-autonomous manner, and CDK6 may be essential for WAT vs BAT lineage commitment. Fig. 6 Re-expression of CDK6 in precursors of KO cells inhibits differentiation towards brown-like adipocytes. a , b , d Representative images of Oil Red O staining of differentiated SVF cells in the presence of BAT inducers ( a ) or WAT inducers ( b , d ). c Representative images of MitoTracker green staining of differentiated SVF cells from iWAT with BAT inducers. MitoTracker green is a cell-permeable probe to label mitochondria. e, g Relative mRNA levels of BAT-specific markers ( e ) and WAT markers ( g ) in the differentiated SVF cells in the presence of BAT or WAT inducers, respectively. Data shown are mRNA fold change normalized to the relative WT controls, which was arbitrarily defined as 1 unit, * p < 0.05, vs WT , t -test ( n = 6). f Immunoblots of the indicated protein levels in differentiated cells from 50 μg of cell lysates. We used α-tubulin as an internal loading control Full size image CDK6 inhibits white fat browning by suppressing RUNX1 in vivo To understand the cellular and molecular mechanisms through which CDK6 negatively regulate white fat browning, we first employed loss of function studies in vivo because of the inverse relationship between CDK6 kinase activity and RUNX1 protein abundance (Figs. 2 l, 4f , 6f , and Supplementary Fig. 3i ). Consistent with previous observation [10] , CDK6 does interact with RUNX1 (Supplementary Fig. 6a, b ), and phosphorylation of RUNX1 on serine 303 was reduced in K43M cells (Supplementary Fig. 6a, b ). Thus, the overabundance of RUNX1 in the absence of CDK6 protein or kinase activity may be due to its reduced phosphorylation status by CDK6 and subsequent reduced degradation. To genetically ablate RUNX1 in WT and K43M mice, we crossed Runx1 fl/fl and K43M;Runx1 fl/fl with Adipoq-Cre mice to remove RUNX1 in mature adipocytes. The presence of DNA recombination of Cdk6 alleles, Cre expression, Runx1 alleles and Floxed- Runx1 alleles, and deleted Floxed- Runx1 alleles were confirmed by PCR [12] , [13] , [31] in adipocytes of the resultant mice (Supplementary Fig. 6c ). Immunoblot analysis demonstrated that the Runx1 −/− and K43M;Runx1 −/− mice still expressed low levels of RUNX1 (Fig. 7f ), which may result from partially penetrant recombination and/or residual RUNX1 protein from progenitors in the adipocytes. Fig. 7 CDK6 inhibits white fat browning by suppressing RUNX1. a Body weight of age-matched male mice (18-week-old) on NCD. * p < 0.05, ( n = 6), vs WT , t -test. ✢ p < 0.05, t -test, K43M;Runx1 −/− vs K43M . b Mass of various fat pads was normalized to body weight of male mice on NCD at 18 weeks of age. No significant changes were observed in the masses of BAT and livers among mice indicated under NCD. Data shown are mean ± S.E. ( n = 10 for each group), * p < 0.05, t -test, vs WT . ✢ p < 0.05, t -test, K43M;Runx1 −/− vs K43M . c GTT after 18 weeks on NCD. d ITT after 18 weeks on NCD. For c and d , n = 10 for each group, * p < 0.05, t -test, K43M vs WT , ♦ p < 0.05, t -test, Runx1 vs WT , ✢ p < 0.05, t -test, K43M;Runx1 −/− vs K43M , ◆ p < 0.05, t -test, K43M;Runx1 −/− vs WT . e Relative mRNA expression levels of BAT-specific markers and WAT-specific markers of iWAT tissues. Data shown are fold changes of mRNA normalized to the control WT , which is arbitrarily set to 1 unit. * p < 0.05 ( n = 6), vs WT control, t -test. ✢ p < 0.05, t -test, K43M;Runx1 −/− vs K43M . f Immunoblots of the indicated protein levels in iWAT from 50 μg of cell lysates of the mice indicated at 18 weeks of age. α-Tubulin is used as an internal loading control. g Ex vivo oxygen consumption of iWAT homogenates from mice indicated. Data are expressed as mean ± S.E., * p < 0.05, vs K43M , t -test. ✢ p < 0.05, t -test, K43M;Runx1 −/− vs K43M . See also Supplementary Figs. 6 and 7 Full size image Compared to K43M mice under both NCD (Fig. 7 ) and HFD ( Supplementary Fig. 7 ), loss of Runx1 in the K43M mice resulted in significantly more body weight and fat masses (Fig. 7a, b and Supplementary Fig. 7a, b ), reversed white fat browning (Supplementary Fig. 6d–g ), and reduced glucose tolerance (Fig. 7c and Supplementary Fig. 7c ). Interestingly, insulin sensitivity was reduced in K43M;Runx1 −/− mice under HFD (Supplementary Fig. 7d ) but not under NCD (Fig. 7d ). Consistent with observed phenotypes, K43M;Runx1 −/− mice had reduced expression of BAT-specific genes and proteins (Fig. 7e, f , Supplementary note) increased WAT-specific genes (Fig. 7e and Supplementary Fig. 7e ), and reduced O 2 consumption (Fig. 7g ). In comparing WT and K43M;Runx1 −/− mice, the similar expression levels of BAT-specific genes and parallel increase in expression of Ap2 and AdipoQ (Fig. 7e ) may in part explain why K43M;Runx1 −/− mice have greater fat pad masses than WT mice. In contrast, loss of Runx1 in WT mice did not affect the gross and histological appearance of subcutaneous fat (Supplementary Fig. 6d–g ), fat pad masses (Fig. 7b and Supplementary Fig. 7b ), cell sizes (Supplementary Fig. 6f ), and UCP-1 staining (Supplementary Fig. 6g ). Similarly, ablation of Runx1 in WT mice also led to increased BAT-specific genes in iWAT (Fig. 7e ). However, these increases are counteracted at least in part by increased WAT-specific genes in iWAT (Fig. 7e ), thus maintaining the homeostatic WAT development. Together, these data demonstrate that RUNX1 mediated the effects of K43M on the regulation of white fat browning. Loss of RUNX1 in K43M precursors reverse white fat browning In vitro, after retroviral infection with MigR1-GFP (GFP) or MigR1-GFP-CRE [17] (GFP-CRE), reduction of RUNX1 in the cells was confirmed by using western blotting (Supplementary Fig. 8a, b , and Fig. 8f ). Compared to those K43M cells ( K43M;Runx1 fl/fl + GFP or K43M + GFP-CRE) (Fig. 8a, b, e, f ), K43M;Runx1 −/− ( K43M;Runx1 fl/fl + GFP-CRE) exhibited reduced BAT differentiation with BAT inducers (Fig. 8c, e, f ), but increased WAT differentiation with WAT inducers (Fig. 8d, g ). By contrast, Runx1 −/− ( Runx1 fl/fl + GFP-CRE) cells and WT cells had comparable capacity of differentiation (Supplementary Fig. 8c, d ). Together, these data suggest that loss of RUNX1 in K43M precursors reversed the phenotypes observed in K43M mutant cells such that the cells displayed increased WAT formation while simultaneously decreasing BAT formation. Fig. 8 Ablation of RUNX1 in K43M precursors inhibits differentiation towards brown-like adipocytes but promotes differentiation towards white adipocytes. a–d Fluorescent photomicrographs of differentiated cells from K43M cells ( K43M;Runx1 fl/fl + GFP or K43M + GFP-CRE) ( a , b ) or K43M;Runx1 −/− ( K43M;Runx1 fl/fl + GFP-CRE)(cd) in the presence of BAT ( a , c ) or WAT inducers ( b , d ). Red fluorescence indicates the Oil Red O staining. Green fluorescence indicates the expression of GFP/GFP-Cre. The yellow fluorescence indicates merged images from red and green fluorescence. Scale bar: 50 μm. e , g Relative mRNA levels of BAT or WAT markers in differentiated cells in the presence of BAT ( e ) or WAT inducers ( g ). Data shown are the mRNA fold change of different mutants normalized to their relative WT controls, which was arbitrarily defined as 1 unit, * p < 0.05, vs WT, t -test ( n = 6). ✢ p < 0.05, t -test, K43M;Runx1 −/− vs K43M . f Immunoblots of the indicated protein levels in the differentiated cells from 50 μg of cell lysates after 7 days in the presence of BAT inducers. α-Tubulin is used as an internal loading control. See also Supplementary Figs. 8 and 9 Full size image RUNX1 binds to mouse Ucp-1 and Pgc-1α promoters To understand the mechanism underline RUNX1-mediated browning, we employed a chromatin immunoprecipitation (CHIP) assay to determine if RUNX1 binds to RUNX1-consensus-binding sites in the mouse Ucp-1 and Pgc-1α genes. Bioinformatic (Matinspector) analysis (Supplementary Fig. 9a, b ) identified three core consensus sequences (TGTGNNN, whereby NNN can stand for TTT or TCA) on the proximal promoter regions of Pgc-1α and Ucp-1 genes, respectively. 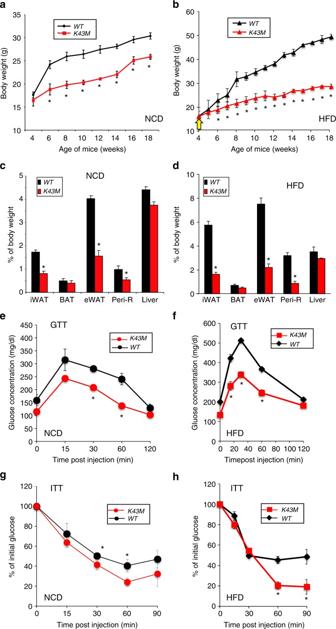Fig. 1 Loss of CDK6 kinase activity in mice leads to an improved metabolic profile.a,bBody weight of age-matched male mice on NCD (a) or HFD (b) for a 14-week observation time. HFD commenced at 4 weeks of age.c,dMass of various fat pads was normalized to body weight of male mice on NCD (c) or HFD (d) at 18 weeks of age. No significant changes were observed in the masses of BAT and livers betweenWTandK43Mmice under NCD and HFD.e,fGTT after 14 weeks on NCD (e) or HFD (f).g,hITT after 14 weeks on NCD (g) or HFD (h). Fora–h, data shown are mean ± S.E. (n= 10 for each group), *p< 0.05,t-test, vsWT. See also Supplementary Figs.2and3 We used both RUNX1- and CDK6-specific antibodies followed by quantitative PCR (qPCR) assay utilizing primers flanking the core consensus sequence (Supplementary Table 1 and Supplementary Fig. 9a, b ). ChIP analysis demonstrated that RUNX1 bound specifically to the sites of Pgc-1α and Ucp-1 genes in WT pre-adipocytes and differentiated adipocytes, and this binding was significantly increased in K43M cells (Supplementary Fig. 9c–e ). These results indicate that increased RUNX1 protein and DNA-binding activity are integral for upregulation of BAT markers in K43M mice. The main finding of this study is that CDK6 is a crucial negative regulator of white to beige fat transition. We provided biochemical and physiological data demonstrating that CDK6, and more specifically its kinase domain, is critical for adipocyte biology and metabolism. We report that genetic inhibition of CDK6 signaling in mice promotes the expression of genes critical for beige cell biogenesis and is associated with browning of WAT, which together impart an advantageous metabolic profile. Our data revealed a previously unknown function of CDK6 in fat metabolism, and suggest that inhibitors of the kinase activity of CDK6 would be beneficial in reversing deleterious effects of metabolic syndromes, and therefore serve as a novel therapeutic target in the treatment of obesity and its related metabolic diseases. We found that CDK6 deficient-mediated WAT browning is due to cell-autonomous effect of CDK6 loss on fat precursor differentiation and conversion of mature white adipocytes, but not due to SNS activation, supporting previous hypothesis that beige cell development is caused by both de-novo differentiation of precursor cells [32] and by transdifferentiation of existing white adipocytes [33] . The browning-mediated by loss of CDK6 kinase activity is physiological relevance since loss of CDK6/kinase activity in mice resulted in weight loss, enhanced energy expenditure, improved glucose tolerance, and insulin sensitization. Conversely, re-expression of CDK6 in mature adipocytes ( WT-A) reverses the beneficial metabolic effects observed in KO mice, indicating that the CDK6 kinase activity regulates metabolic homeostasis in a cell-autonomous manner, although whether this is due to the appearance of brite fat or whether other mechanisms play a role is difficult to discern at the moment. We also found that the effects of CDK6 in conversion of fat-storing cells into fat-burning cells is independent of pRB activity and, therefore, most likely independent of cell cycle control. pRB has been show to play multiple roles in metabolic functions including repressing PGC-1 α expression [34] and suppressing peroxisome proliferator-activated receptor gamma subunit [35] . Mouse embryo fibroblasts deficient in pRB did not undergo adipose conversion in response to standard adipogenic inducers, but rather differentiated into brown adipose [36] . We demonstrate that CDK6 has pRB-independent role in adipogenesis by regulating RUNX1, one of the downstream effectors of CDK6 [10] known to be frequently mutated in human leukemia and play a role in hematopoiesis [37] . To the best of our knowledge, our findings demonstrate, for the first time, a molecular interplay between CDK6 and RUNX1 and in the regulation of white fat browning. This mechanism appears, at least in part, to be due to a CDK6 kinase-mediated suppression of RUNX1 that normally promotes Ucp-1 and Pgc-1α expression. Genetic deletion of Runx1 in K43M mice rescues most of the phenotype observed in mutant mice in vivo and restores WAT differentiation capacity of K43M precursors in vitro, demonstrating a downstream role for RUNX1 in CDK6-mediated white fat browning. Mechanistically, our results suggest that CDK6 is integrated into the white fat browning pathways and therefore serve as a sensor and an effector of cellular energy status as shown in Fig. 9 . In response to food intake, increased expression of cyclin D1 [38] and CDK6 (Supplementary Fig. 1 ) leads to activation of CDK6. In addition, the canonical cascade of events is initiated, including the activation of Notch1 [39] and AKT1 [40] . Notch1 activates CDK6 via upregulation of CDK6 and/or by increased cyclin D3 protein [41] . AKT1 activates CDK6 by stabilizing cyclin D2 [42] . Phosphorylation of RUNX1 by CDK6 and other kinases such as ERK and CDK1 [10] promotes RUNX1 proteolytic degradation [10] , resulting in a reduction of RUNX1 recruitment to the proximal promoter regions of Ucp-1 and Pgc-1α (Supplementary Fig. 9 ), subsequently leading to reduced level of BAT-specific protein expression. In the absence of CDK6 protein/kinase activity, RUNX1 is stabilized, BAT-specific protein expression is increased, and obesity and its related metabolic diseases are suppressed. Fig. 9 A working model of the role of CDK6 in negative regulation of white fat browning by suppressing RUNX1. In response to food intake, increased expression of cyclin D1 [38] and CDK6 leads to activation of CDK6 (Supplementary Fig. 1 ). In addition, the canonical cascade of events is initiated, including the activation of Notch1 [39] and AKT1 [40] . Notch1 activates CDK6 via upregulation of CDK6 and/or by increased cyclin D3 protein [41] . AKT1 activates CDK6 by stabilizing cyclin D2 [42] . 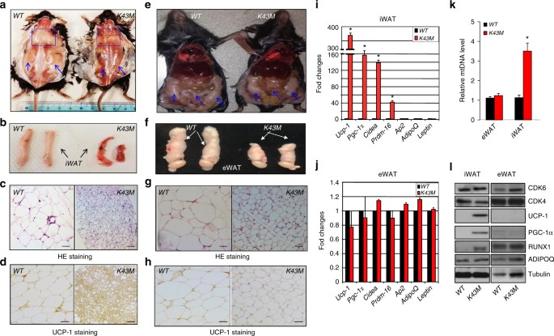Fig. 2 Loss of CDK6 kinase activity in mice induced white fat browning.a,eAppearance of male posterior-subcutaneous WAT (sWAT) (a), and dorsal view of NCD-fedWTandK43Mmice (e), emphasized with blue squares and arrows.b,fAppearance of a close view of the iWAT (b) and eWAT (f) from the mice indicated.c,gRepresentative light microscopic images of H&E-stained sections of iWAT (n= 6) and eWAT (n–6) from male mice indicated (scale bars: 100 μm).d,hRepresentative images of UCP-1 immunohistochemical staining (n= 6) of iWAT and eWAT from mice indicated at 18 weeks of age (scale bars: 100 μm).i,jRelative mRNA expression levels of BAT-specific markers (Ucp-1,Pgc-1α,Cidea, andPrdm16)and WAT-specific markers (Ap2,adiponectin-AdipoQ, andLeptin) of iWAT (i) and eWAT (j) tissues fromWTandK43Mmice. Data shown are mRNA fold change normalized to the controlWT, which is arbitrarily set to 1 unit.kRelative expression levels of mtDNA of eWAT and iWAT fromWTandK43Mmice. Data shown are fold change of mtDNA compared to control. Foriandj, *p< 0.05, vsWT(n= 6),t-test.iImmunoblots of the indicated protein levels in iWAT and eWAT from 50 μg of cell lysates ofWTandK43Mmice at 18 weeks of age. α-Tubulin is used as an internal loading control. See also Supplementary Figs.2and3 Phosphorylation of RUNX1 by CDK6 and other kinases such as ERK and CDK1 [10] promotes RUNX1 proteolytic degradation [10] , resulting in a reduction of RUNX1 recruitment to the proximal promoter regions of Ucp-1 and Pgc-1α (Supplementary Fig. 9 ), subsequently leading to reduced level of BAT-specific protein expression. In the absence of CDK6 protein/kinase activity, RUNX1 is stabilized, BAT-specific protein expression is increased, and obesity and its related metabolic diseases are suppressed Full size image Therapeutically, our data also show that CDK6 could be better therapeutic target in metabolic diseases than CDK4, a cyclin-dependent kinase that has been implicated in metabolism by phosphorylating PGC-1α [43] and insulin receptor substrate 2 [44] . However, loss of CDK4 has been shown to result in insulin-deficient diabetes due to a severe decrease in β-cell growth [45] . In contrast, loss of function of CDK6 enhances both energy expenditure and improves glucose tolerance and insulin sensitivity, but has no obvious effect on pancreas [46] . Thus, inhibition of CDK6 kinase activity might open up new perspectives in the control of metabolic diseases and could be a better therapeutic target in obesity-related metabolic diseases such as type II diabetes. Overall, our findings reveal that CDK6 kinase activity functions as a potent regulator of white to beige cell transition, providing a new therapeutic target for pharmacological intervention aimed at combatting the imminent obesity epidemic and its related metabolic diseases. Mice Generation of different mature adipocytes-specific mutant mice and K43M;Runx1 −/− mice We backcrossed mice bearing the WT-LSL and K43M-LSL (we made) alleles eight times to C57BL/6. Mature adipocyte-specific WT-A/K43M-A mutant mice, Runx1 −/− mice, and K43M;Runx1 −/− mice were produced by crossing WT-LSL , K43M-LSL , Runx1 fl/fl (Jackson lab, stock number: 010673) and K43M;Runx1 fl/fl alleles with Adipoq-Cre mice (Jackson lab, stock number: 010803), respectively. All experiments were performed according to the guidelines of the Institutional Animal Care and Use Committee of Tufts University. GTT and ITT tests The experimental procedures described previously [47] . We used mice at age of 12–18 weeks. Body composition Body composition was analyzed by NMR. Energy expenditure, locomotor activity, and food intake Energy expenditure, locomotor activity, and food intake were determined by metabolic cages using a TSE system. Both NMR and TSE system are in the Adipocyte Biology and Nutrient Metabolism Core of BNORC. Oxygen consumption (VO 2 ), carbon dioxide production (VCO 2 ), and spontaneous motor activity during 3 consecutive days were measured and normalized to lean mass. Ex vivo oxygen consumption Direct ex vivo tissue oxygen consumption was measured by a Clark electrode (Strathkelvin Instruments in Dana-Farber). Freshly isolated fat tissue was minced in respiration buffer (1.5 mM pyruvate, 25 mM glucose, 2% bovine serum albumin) and placed in electrode chambers. The O 2 consumption rate was normalized to tissue weight. In vitro differentiation assay The primary ADSCs from the SVF of iWAT of WT , KO / K43M , Runx1 fl/fl , and K43M;Runx1 fl/fl mice were isolated as previously described [48] . To re-express CDK6 or delete RUNX1, KO/Runx1 fl/fl / K43M;Runx1 fl/fl were infected with MigR1-GFP-CRE [17] . In order to induce differentiation, adipocyte progenitor cells were left for a further 48 h after reaching confluence, then induced with white [49] or brown/beige adipocytes inducers [50] for 7 days. On day 8, accumulation of lipid-containing cells was detected by Oil red O staining as described [51] . Fluorescent photomicrographs of differentiated cells were presented. Red fluorescence indicates the Oil-Red-O staining. Green fluorescence indicates the expression of GFP/GFP-Cre. Yellow fluorescence indicates the merged Red and Green fluorescence. In a subset of experiments, the differentiated cells were also stained with MitoTracker, a cell-permeable probe used to label mitochondria. Adipogenic gene expression of WAT and BAT markers was analyzed by reverse transcription PCR (RT-PCR) and immunoblotting. Chromatin immunoprecipitation We performed ChIP according to the protocol described by Upstate Biotechnology. Pre-adipocytes and differentiated cells were treated with formaldehyde and immunoprecipitated with antibody against RUNX1 ( rabbit anti-RUNX1 antibody , Cat. ab23980 ) , CDK6 (C-21, Santa Cruz), and normal rabbit IgG, respectively. The immunoprecipitates were eluted and reverse crosslinked for 5 h at 65 °C. qPCR was performed with the primers listed in Supplemental Table 1 (site 1-site 3 of Ucp-1 and Pgc-1α ). For the internal control, genomic DNA was extracted from pre-adipocytes or differentiated cells and 1% (input) of the extracted DNA was amplified with the same primers listed in Supplemental Table 1 . Immunoblotting, IP-Western, and RNA purification Mice were sacrificed by CO 2 and spinal dislocation, and tissue samples were removed, clamp-frozen in liquid nitrogen, and stored at −80 °C until being processed as described previously [12] , [13] . Antibodies used in this study included CDK6 (ab3126, mouse monoclonal antibody, Abcam), CDK6 (C-21, Santa Cruz, 1:1000 dilution), RUNX1 (Ab23980, Rabbit polyclonal antibody, 1:1000 dilution, Abcam), CDK4 (C-22, Santa Cruz, 1:1000 dilution), RUNX1-phospho-S303 (Ab55308, Abcam, 1:1000 dilution), α-Tubulin (Sigma, mouse monoclonal, 1:2000 dilution), UCP-1 (AB23841, Abcam, 1:1000 dilution), PGC-1α (SC13067, H-300, Santa Cruz, 1:1000 dilution), Anti-Tyrosine Hydroxylase antibody (ab75875, 1:1000 dilution). For Supplementary Fig. 6a , we immunoprecipitated RUNX1 with antibody (AB54869-100, mouse monoclonal antibody, Abcam) from extracts of adipose tissues of iWAT and probed the blots with the indicated antibodies RUNX1-phospho-S303 (Ab55308, Abcam), CDK6 (C-21, Santa Cruz), and total RUNX1 (Ab23980, Rabbit polyclonal antibody, Abcam). For Supplementary Fig. 6b , we immunoprecipitated CDK6 with antibody (ab3126, mouse monoclonal antibody, Abcam) from extracts of adipose tissues of iWAT and probed the blots with the same antibodies described above as for Supplementary Fig. 6a . For detecting CDK6, we used CDK6 (C-21, Santa Cruz). The antibody used for CHIP assay was obtained from Abcam (rabbit anti-RUNX1 antibody, Cat. ab23980). Quantitative real-time PCR (RT-PCR) The experimental procedures are same as those described previously [47] . 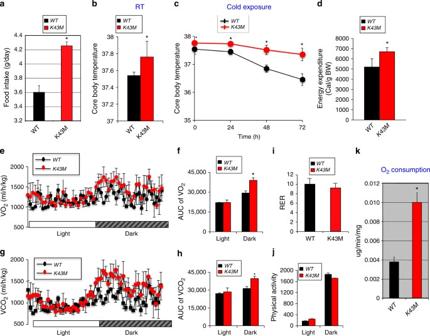Fig. 3 Loss of CDK6 kinase activity in mice leads to increased food intake, body temperature, adaptability to cold exposure and energy expenditure.aBar graphs demonstrating food intake of age-matched maleWTandK43Mmice at 18 weeks of age.b,cCore body temperature of male mice at room temperature (b, RT) or at 4 °C (c) for up to 72 h (n= 6 per group).dEnergy expenditure (EE) was calculated based on the formula below: EE = (3.815 + 1.232 × RER) x VO2/lean mass (g). Fora–d, data are expressed as mean ± S.E., *p< 0.05, vsWT,t-test.e–h, Oxygen consumption (VO2) (e, f) and CO2production (VCO2) (g, h) from metabolic cages of maleWTandK43Mmice on NCD (n= 6) in 12 h light and dark phases. VO2and VCO2were normalized by lean mass. *p< 0.05, vsWT, log-rank tests.iBar graphs displaying mean Respiratory Exchange Ratios (RER) over 24-h period. RER was calculated as the volume of CO2vs the volume of oxygen (VCO2/VO2).jPhysical activity of maleWTandK43Mmice in the periods of 12 h light and 12 h dark phase.kEx vivo oxygen consumption of iWAT homogenates from differentWTandK43Mmice. Data are expressed as mean ± S.E., *p< 0.05, vsWT,t-test The 36B4 gene, encoding an acidic ribosomal phosphoprotein P0 (RPLP0), was used as an invariant internal control. The Primer sequences for genotyping of Cdk6 mutant [12] , [13] and Runx1 mutant mice [31] , for RT-PCR of brown fat genes including Ucp-1 , Pgc-1α , Cidea , and Prdm16 (ref. [47] ) are same as those described previously. Other primer sequences for RT-PCR or for qPCR are listed in Supplemental Table 1 . Statistical methods and statistical analysis For most experiments, the sample size was chosen based on expected differences between experimental and control groups in order to provide adequate power to detect a significant difference specifying α = 0.05, two-tailed testing, and power (=1− β ) of 80%, using commercially available software packages (Statistical Solutions nQuery Advisor; http://www.statsol.ie/nquery/nquery.htm ). 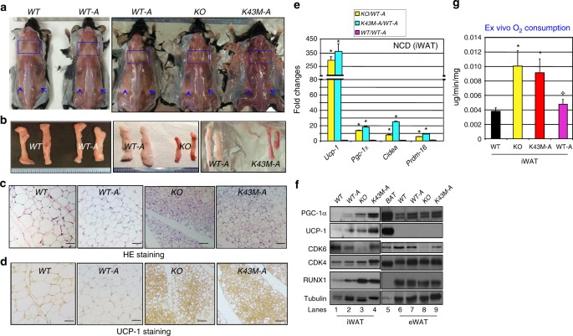Fig. 4 Re-expression of CDK6 in mature adipocytes ofKOmice reverses white fat browning. Loss of kinase activity in mature adipocytes preserves the effect of loss of kinase activity in germline on white fat browning.aAppearance of male (18 weeks of age) posterior-sWAT of NCD-fedWT,WT-A,KO, andK43M-A, emphasized with blue squares and arrows.bAppearance of isolated iWAT from the mice indicated ina.cRepresentative light microscopic images of H&E-stained sections of iWAT (n= 6) from male (18 weeks of age) mice indicated ina(scale bars: 100 μm).dRepresentative images of UCP-1 staining (n= 6) of iWAT from mice indicated at 18 weeks of age (scale bars: 100 μm).eRelative mRNA expression levels of BAT-specific markers (Ucp-1,Pgc-1α,Cidea, andPrdm16)of iWAT under NCD. Data shown are mRNA fold change normalized to their respective controls,WTorWT-A. *p< 0.05,n= 6,t-test, comparing experimental group vs its control.fImmunoblots of the indicated protein levels in iWAT and eWAT from 50 μg of cell lysates. Twenty micrograms of cell lysates of BAT was used as a positive control for UCP-1 and PGC-1α, and α-tubulin was utilized as an internal loading control.gEx vivo oxygen consumption of iWAT homogenates from mice. Data are expressed as mean ± S.E., *p< 0.05,n= 6, vsWT,t-test.✢p< 0.05,n= 6 vsKO,t-test. See also Supplementary Figs.3and5 All data are expressed as means ± S.E. We calculated statistical significance using Student’s t -test, or log-rank tests, with P < 0.05 considered significant. 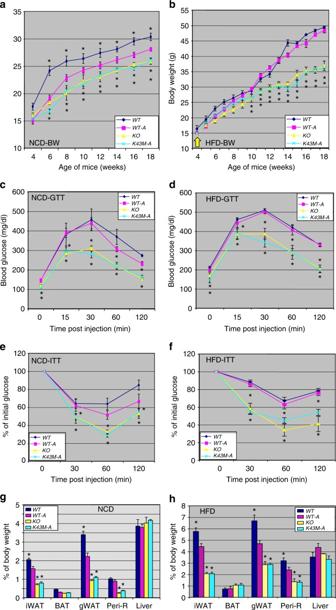Fig. 5 Re-expression of CDK6 in mature adipocytes reversed the beneficial metabolic effects observed inKOmice, whereas re-expression of kinase dead CKD6 recapitulates this metabolic profile.a,bBody weight of age-matched male mice on NCD (a) or HFD (b) for 14-week observation time. HFD started at age of 4 weeks.c,dGTT after 18 weeks on NCD (c) or HFD (d).e,fITT after 18 weeks on NCD (e) or HFD (f).g,hMass of various fat pads was normalized to body weight of male mice on NCD (g) or HFD (h) at age of 18 weeks. No significant changes were observed in the masses of BAT and livers in those mice under NCD and HFD. Fora–h, data are expressed as mean ± S.E. (n= 10 for each group), *p< 0.05,t-test, vsWT-A. See also Supplementary Fig.3 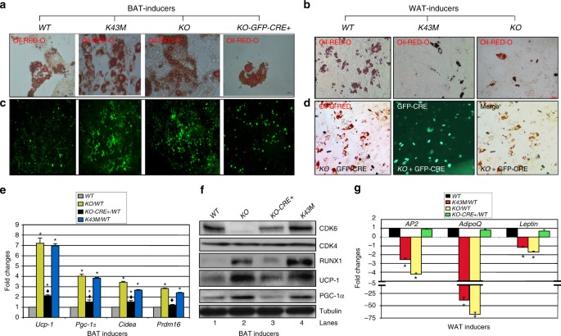Fig. 6 Re-expression of CDK6 in precursors ofKOcells inhibits differentiation towards brown-like adipocytes.a,b,dRepresentative images of Oil Red O staining of differentiated SVF cells in the presence of BAT inducers (a) or WAT inducers (b,d).cRepresentative images of MitoTracker green staining of differentiated SVF cells from iWAT with BAT inducers. MitoTracker green is a cell-permeable probe to label mitochondria. e,gRelative mRNA levels of BAT-specific markers (e) and WAT markers (g) in the differentiated SVF cells in the presence of BAT or WAT inducers, respectively. Data shown are mRNA fold change normalized to the relativeWTcontrols, which was arbitrarily defined as 1 unit, *p< 0.05, vsWT,t-test (n= 6).fImmunoblots of the indicated protein levels in differentiated cells from 50 μg of cell lysates. We used α-tubulin as an internal loading control 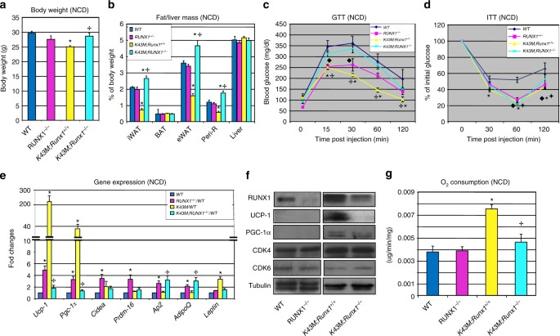Fig. 7 CDK6 inhibits white fat browning by suppressing RUNX1.aBody weight of age-matched male mice (18-week-old) on NCD. *p< 0.05, (n= 6), vsWT,t-test.✢p< 0.05,t-test,K43M;Runx1−/−vsK43M.bMass of various fat pads was normalized to body weight of male mice on NCD at 18 weeks of age. No significant changes were observed in the masses of BAT and livers among mice indicated under NCD. Data shown are mean ± S.E. (n= 10 for each group), *p< 0.05,t-test, vsWT.✢p< 0.05,t-test,K43M;Runx1−/−vsK43M.cGTT after 18 weeks on NCD.dITT after 18 weeks on NCD. Forcandd,n= 10 for each group, *p< 0.05,t-test,K43MvsWT,♦p< 0.05,t-test,Runx1vsWT,✢p< 0.05,t-test,K43M;Runx1−/−vsK43M,◆p< 0.05,t-test,K43M;Runx1−/−vsWT.eRelative mRNA expression levels of BAT-specific markers and WAT-specific markers of iWAT tissues. Data shown are fold changes of mRNA normalized to the controlWT, which is arbitrarily set to 1 unit. *p< 0.05 (n= 6), vsWTcontrol,t-test.✢p< 0.05,t-test,K43M;Runx1−/−vsK43M.fImmunoblots of the indicated protein levels in iWAT from 50 μg of cell lysates of the mice indicated at 18 weeks of age. α-Tubulin is used as an internal loading control.gEx vivo oxygen consumption of iWAT homogenates from mice indicated. Data are expressed as mean ± S.E., *p <0.05, vsK43M,t-test.✢p< 0.05,t-test,K43M;Runx1−/−vsK43M. See also Supplementary Figs.6and7 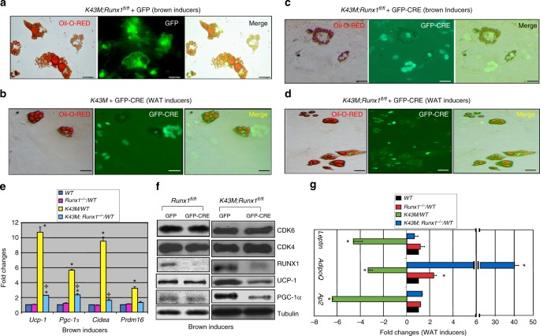Fig. 8 Ablation of RUNX1 inK43Mprecursors inhibits differentiation towards brown-like adipocytes but promotes differentiation towards white adipocytes.a–dFluorescent photomicrographs of differentiated cells fromK43Mcells (K43M;Runx1fl/fl+ GFP orK43M+ GFP-CRE) (a,b) orK43M;Runx1−/−(K43M;Runx1fl/fl+ GFP-CRE)(cd) in the presence of BAT (a,c) or WAT inducers (b,d). Red fluorescence indicates the Oil Red O staining. Green fluorescence indicates the expression of GFP/GFP-Cre. The yellow fluorescence indicates merged images from red and green fluorescence. Scale bar: 50 μm.e,gRelative mRNA levels of BAT or WAT markers in differentiated cells in the presence of BAT (e) or WAT inducers (g). Data shown are the mRNA fold change of different mutants normalized to their relativeWTcontrols, which was arbitrarily defined as 1 unit, *p< 0.05, vs WT,t-test (n= 6).✢p< 0.05,t-test,K43M;Runx1−/−vsK43M.fImmunoblots of the indicated protein levels in the differentiated cells from 50 μg of cell lysates after 7 days in the presence of BAT inducers. α-Tubulin is used as an internal loading control. See also Supplementary Figs.8and9 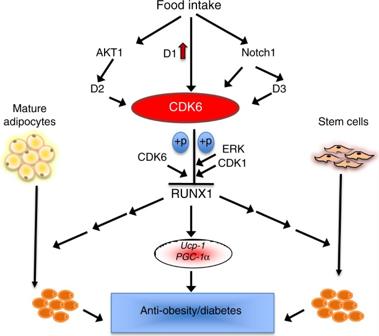Fig. 9 A working model of the role of CDK6 in negative regulation of white fat browning by suppressing RUNX1. In response to food intake, increased expression of cyclin D138and CDK6 leads to activation of CDK6 (Supplementary Fig.1). In addition, the canonical cascade of events is initiated, including the activation of Notch139and AKT140. Notch1 activates CDK6 via upregulation of CDK6 and/or by increased cyclin D3 protein41. AKT1 activates CDK6 by stabilizing cyclin D242. Phosphorylation of RUNX1 by CDK6 and other kinases such as ERK and CDK110promotes RUNX1 proteolytic degradation10, resulting in a reduction of RUNX1 recruitment to the proximal promoter regions ofUcp-1andPgc-1α(Supplementary Fig.9), subsequently leading to reduced level of BAT-specific protein expression. In the absence of CDK6 protein/kinase activity, RUNX1 is stabilized, BAT-specific protein expression is increased, and obesity and its related metabolic diseases are suppressed Data availability All relevant data are available from the authors.